Phonon localization drives polar nanoregions in a relaxor ferroelectric Relaxor ferroelectrics exemplify a class of functional materials where interplay between disorder and phase instability results in inhomogeneous nanoregions. Although known for about 30 years, there is no definitive explanation for polar nanoregions (PNRs). Here we show that ferroelectric phonon localization drives PNRs in relaxor ferroelectric PMN-30%PT using neutron scattering. At the frequency of a preexisting resonance mode, nanoregions of standing ferroelectric phonons develop with a coherence length equal to one wavelength and the PNR size. Anderson localization of ferroelectric phonons by resonance modes explains our observations and, with nonlinear slowing, the PNRs and relaxor properties. Phonon localization at additional resonances near the zone edges explains competing antiferroelectric distortions known to occur at the zone edges. Our results indicate the size and shape of PNRs that are not dictated by complex structural details, as commonly assumed, but by phonon resonance wave vectors. This discovery could guide the design of next generation relaxor ferroelectrics. Understanding the development of inhomogeneous nanoregions is a scientific challenge at the heart of many technologically important materials, including relaxor ferroelectrics, colossal magnetoresistance maganites, diluted magnetic semiconductors and some superconductors [1] . Relaxor ferroelectrics [2] in particular exhibit a large electromechanical response that makes them useful in medical ultrasonics, military sonar and has potential for future-generation actuators and motors [3] , [4] , [5] . Burns and Dacol [6] proposed polar nanoregions PNRs and the upper temperature of their stability range, the Burns temperature ( T d ), to explain changes in the optical index of refraction and the onset of relaxor behaviour, which occurs several hundred degrees above the Curie temperature, T C . The existence of PNRs has been supported by neutron scattering [7] , nuclear magnetic resonance [8] and piezoresponse force microscopy [9] , but cold-neutron diffuse scattering [10] and dynamical pair distribution function [11] experiments indicate that PNRs fluctuate at T d and do not become static until below an intermediate temperature between T C and T d . Bosak et al. [12] did three-dimensional (3D) mappings of the PNR diffuse scattering and found that they could be described in terms of transverse-wave-like distortions. The large electromechanical response of relaxors was explained by an instability in the transverse acoustic (TA) phonon induced by reorienting PNRs [13] . It was speculated that the ‘waterfall’ effect, where the transverse optic (TO) phonon dispersion curve forms a vertical column near the zone centre, may be caused by PNRs [14] , but this explanation did not hold up against more quantitative mode-coupling models [15] and observations that the ‘waterfall’ effect occurs even without PNRs [16] . Recently, Swainson et al. [17] found similar soft phonon columns near the zone edges in PMN ((Pb(Mg 1/3 Nb 2/3 )O 3 ) and attributed them to competing antiferroelectric distortions [17] . The extreme slow down of fluctuating PNRs on cooling has been explained in terms of quenched random electric fields [18] , [19] , but a connection to the lattice dynamics is unclear since the mass inertia of the polar displacements is not included in these models. Furthermore, Sherrington [20] recently suggested that since the dilution of the random field with increasing PT in PMN- x PT ((Pb(Mg 1/3 Nb 2/3 )O 3 ) 1− x -(PbTiO 3 ) x ) does not decrease the relaxor onset temperature, random fields may play only a secondary role in relaxor behaviour. It has also been argued that PNRs are chemically ordered nanoregions [21] , but not all relaxors exhibit chemical order and electron diffraction has indicated that PNRs are not caused by chemical order [22] . Hirota et al. [23] argued that in addition to being polarized, PNRs must also have an offset displacement along the polarization direction. More recently it has been suggested that formation of PNRs may result from a phase transition to a vortex state [24] . The formation and the slowing of PNRs has been explained in terms of defect-pinned intrinsic localized modes (ILMs)—also known as discrete breathers [25] , [26] , [27] . While ILMs are spatially localized nonlinear excitations that occur in perfect crystals [28] , [29] , [30] , in this model a local enhancement of the nonlinearity associated with off-centring Pb atoms [31] instigates the formation of ILMs on cooling [25] , [26] , [27] . The ILM frequency then slows below that of the TO phonon into the frequency gap between the TA and TO phonons, and eventually vanishes as PNRs become static [25] , [26] , [27] . There is an additional phonon localization mechanism for disordered systems; coherent multiple scattering interference from random, strongly scattering sites can produce localized regions of trapped standing waves—an effect known as Anderson localization [32] , [33] , [34] , [35] . Originally proposed to explain the localization of electron wavefunctions in disordered materials [32] , Anderson localization has since been observed for a variety of systems ranging from ultrasound in an elastic network [33] to ultra cold atoms [34] , [35] , but it has not been observed for phonons. In this article, neutron scattering results indicate that a narrow band of Anderson-localized ferroelectric TO phonons develops in PMN-30%PT with the onset of strong scattering from disordered resonance modes forming near T d . Additional resonances and phonon localization at the zone edges explain the competing zone-edge antiferroelectric distortions observed in PMN [17] . The resulting single-wavelength-trapped ferroelectric standing phonons, slowed by nonlinearity, explain the PNRs and relaxor properties. That the size and shape of PNRs, as well as the positions in the zone of the both ferroelectric and antiferroelectric distortions (structure factors), can be explained by the interaction of a single preexisting resonance mode with the TO phonon dispersion surface, and that the precursor resonance mode is observed 200 K above the stability limit of the structural PNRs, all lead us to conclude that the phonon localization drives the PNRs. 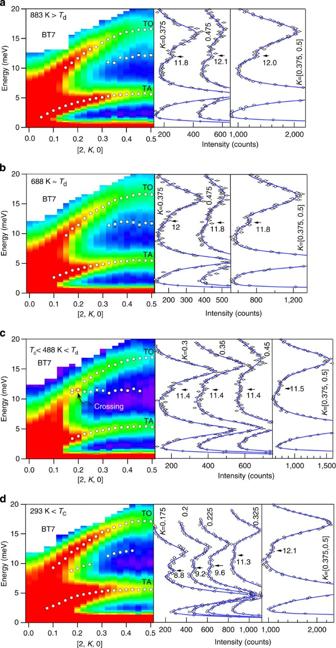Figure 1: Phonons measured using a triple-axis spectrometer. (a) On left, spectrum measured using the BT7 triple-axis spectrometer alongQ=[2,K, 0] at 883 K, which is a temperature well above the Burns temperature (Td≈680 K). The open circles indicate the peak positions from fits to the TA and TO modes and a weaker mode inbetween. Panels on the right side show fits to the modes in the neutron spectrum at a few values ofKand integratedK=[0.375, 0.5], with data offset in intensity for clarity. (b) The same spectrum and fits measured at 688 K, nearTd. (c) Spectrum at 488 K, a temperature betweenTCandTd. A resonant crossing with the TO and the weaker mode is indicated atK=0.2. (d) Spectrum at 293 K, a temperature belowTC. Uncertainties are statistical and represent one s.d. Triple-axis inelastic neutron scattering Figure 1 shows an extra mode between the TA and TO phonons in the temperature-dependent phonon dispersion of PMN-30%PT. These triple-axis neutron scattering measurements were taken in transverse geometry along neutron momentum transfer Q =[2, K , 0], for K =[0, 0.5]. At 883 K ( Fig. 1a ), about 200 K above T d (≈680 K, see Supplementary Fig. 1 ), the extra mode is located below the TO phonon, intersecting the zone boundary at 12.0±0.1 meV. Its integrated intensity represents 6±0.4% of the TO branch for a K =[0.375, 0.5] integration. This extra mode is not accounted for by the average long-range crystal structure, and the limited dependence of its energy on wave vector suggests that it is partially localized. On cooling to 688 K (near T d ), this extra mode becomes completely dispersionless, demonstrating that it becomes well localized ( Fig. 1b ). As measured in the range K =[0.375, 0.5], the localizing mode also loses some intensity relative to the TO mode from 6 to 4.5±0.8% and softens slightly from 12 to 11.8±0.1 meV ( Fig. 1b ). On further cooling to 488 K ( Fig. 1c ), which is in between T d and T C (about 400 K), the mode remains dispersionless (localized) as it softens to 11.5±0.2 meV, but its intensity shifts away from the zone boundary towards the TO mode. The local mode intensity diminishes to 1.3±0.3% of the TO intensity integrated in the range K =[0.375, 0.5], but becomes enhanced near the resonant crossing with the TO mode at K =0.2, indicated in Fig. 1c . As shown in Fig. 2a , at the resonant crossing ( K =0.2) the peaks exhibit a lineshape that fits a sharp peak (localized mode) superimposed on a broader peak (TO mode). Unlike the avoided crossing effects often observed with resonant local modes [36] , the TO mode exhibits no break at the crossing. For K =0.15 and lower, the TO mode becomes overdamped and the localizing mode intensity becomes weak. The 688 K spectrum, Fig. 2b , is qualitatively different, and the localizing mode, which has a constant intensity for K >0.3, is not evident below K =0.3. There is also an additional intensity bridging the gap between the TA and TO modes, which may be evidence of a ‘waterfall’ effect [14] , although this disappears at 488 K. On cooling to 293 K ( Fig. 1d ), below T C , the localizing mode develops strong dispersion (delocalizes). This mode delocalization coincides with the growth of the PNRs into larger domains [7] . Additional supporting measurements and analysis confirming the localizing mode are described in Supplementary Figs 2–4 . Figure 1: Phonons measured using a triple-axis spectrometer. ( a ) On left, spectrum measured using the BT7 triple-axis spectrometer along Q =[2, K , 0] at 883 K, which is a temperature well above the Burns temperature ( T d ≈680 K). The open circles indicate the peak positions from fits to the TA and TO modes and a weaker mode inbetween. Panels on the right side show fits to the modes in the neutron spectrum at a few values of K and integrated K =[0.375, 0.5], with data offset in intensity for clarity. ( b ) The same spectrum and fits measured at 688 K, near T d . ( c ) Spectrum at 488 K, a temperature between T C and T d . A resonant crossing with the TO and the weaker mode is indicated at K =0.2. ( d ) Spectrum at 293 K, a temperature below T C . Uncertainties are statistical and represent one s.d. 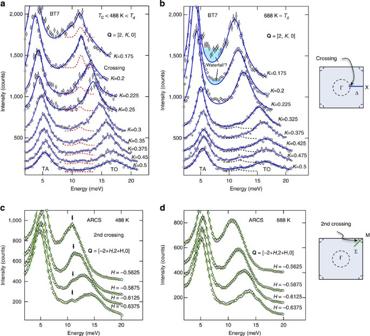Figure 2: Phonon spectrum measured near resonant crossings. (a) Fits to the triple-axis (BT7) spectrum measured at 488 K for the crossing near the Γ point along Γ to X in the (200) zone (path is indicated in illustration to the right), where the red dashed-line peaks correspond to the fits to the local mode. (b) Fits to the spectrum measured at 688 K along the same Γ to X path, where the black dashed-line peaks correspond to the fits to the local mode. The blue shaded area indicates extra intensity not accounted for by the peak fit, which may correspond to a ‘waterfall’ effect associated with mode coupling, see text. (c) Fits to the time-of-flight chopper (ARCS) spectrum measured at 488 K along Γ to M in the (10) zone (the path is indicated in the illustration on the right). The arrows indicate an extra dispersionless peak superimposed on the TO mode. (d) Fits to the ARCS spectrum measured at 688 K along the same Γ to M path. Full size image Figure 2: Phonon spectrum measured near resonant crossings. ( a ) Fits to the triple-axis (BT7) spectrum measured at 488 K for the crossing near the Γ point along Γ to X in the (200) zone (path is indicated in illustration to the right), where the red dashed-line peaks correspond to the fits to the local mode. ( b ) Fits to the spectrum measured at 688 K along the same Γ to X path, where the black dashed-line peaks correspond to the fits to the local mode. The blue shaded area indicates extra intensity not accounted for by the peak fit, which may correspond to a ‘waterfall’ effect associated with mode coupling, see text. ( c ) Fits to the time-of-flight chopper (ARCS) spectrum measured at 488 K along Γ to M in the ( 10) zone (the path is indicated in the illustration on the right). The arrows indicate an extra dispersionless peak superimposed on the TO mode. ( d ) Fits to the ARCS spectrum measured at 688 K along the same Γ to M path. Full size image Time-of-flight inelastic neutron scattering Time-of-flight (TOF) neutron scattering measurements depicted in Fig. 3a,b confirm the mode observed along [100] and also show that it appears at the same energy in the [110] direction ( Fig. 3c,d ). Furthermore, as indicated in Fig. 3c,e,f , a second crossing with the TO mode occurs along the [110] direction near the zone-edge M point. Similar to the crossing near the zone centre ( Figs 1c and 2a ), on cooling from 688 K ( Fig. 3e ) to 488 K ( Fig. 3f ) an intensity enhancement of the local mode occurs at the second crossing, as indicated in Fig. 3f . Figure 2c shows that this spectrum can also be fit by a sharp peak superimposed on the TO peak, but that the intensity enhancement is not as strongly peaked at the second crossing ( Fig. 2c ) as it is at Q =[2, 0.2, 0] ( Fig. 2a ). Interestingly, the M point corresponds to antiferroelectric atomic displacements in the TO phonon, and this is the position where antiferroelectric distortions were identified in PMN [17] . 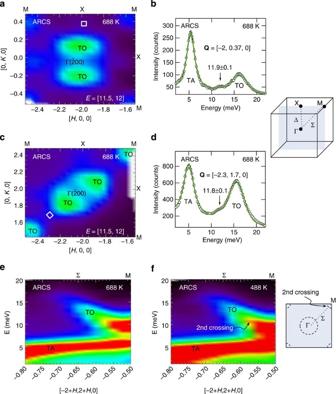Figure 3: Phonons measured using a time-of-flight chopper spectrometer. (a) Intensity slice of the data at 688 K in the (00) zone at the energy of the localizing mode;E=[11.5, 12] meV. Transverse scattering geometry selects the TO mode preferencially alongQ=[0,K, 0] between Γ and X. The locations of the high-symmetry points in the zone are shown on the right of the figures. The small white box indicates the location and theKandHintegration range of the energy cut inb. (b) Energy cut atQ=[−2, 0.37, 0] confirming the localizing mode feature found inFig. 1. (c) Intensity slice of the data in the (20) zone at the energy of the localizing mode with the same energy integration range as ina. The small white box indicates the location and theKandHintegration range of the energy cut ind. (d) Energy cut atQ=[−2.3, 1.7, 0] showing that the localizing mode feature appears along the [110] direction at the same energy as along the [100] direction. (e) Phonon dispersion at 688 K alongQ=[−2+H, 2+H, 0] in the (10) zone. (f) Same ase, except at 488 K. The indicated second crossing is the point where the localizing mode intersects the TO mode near the M point at the zone edge, as illustrated on the right. Figure 3: Phonons measured using a time-of-flight chopper spectrometer. ( a ) Intensity slice of the data at 688 K in the ( 00) zone at the energy of the localizing mode; E =[11.5, 12] meV. Transverse scattering geometry selects the TO mode preferencially along Q =[0, K , 0] between Γ and X. The locations of the high-symmetry points in the zone are shown on the right of the figures. The small white box indicates the location and the K and H integration range of the energy cut in b . ( b ) Energy cut at Q =[−2, 0.37, 0] confirming the localizing mode feature found in Fig. 1 . ( c ) Intensity slice of the data in the ( 20) zone at the energy of the localizing mode with the same energy integration range as in a . The small white box indicates the location and the K and H integration range of the energy cut in d . ( d ) Energy cut at Q =[−2.3, 1.7, 0] showing that the localizing mode feature appears along the [110] direction at the same energy as along the [100] direction. ( e ) Phonon dispersion at 688 K along Q =[−2+ H , 2+ H , 0] in the ( 10) zone. ( f ) Same as e , except at 488 K. The indicated second crossing is the point where the localizing mode intersects the TO mode near the M point at the zone edge, as illustrated on the right. Full size image Analysis of the localizing mode structure The narrow linewidth of the localizing mode at 488 K, Fig. 2a,c , indicates that it remains long lived. As described in more detail in Supplementary Fig. 5 , the localizing mode linewidth gets somewhat narrower as the mode localizes. This is surprising, given that the mode develops resonant crossings with the TO mode ( Figs 1c , 2a,c and 3f ), which would typically generate TO phonons that radiate energy away from the local mode, causing a shortened lifetime (broader linewidth), but there is an alternative scenario. The lifetime broadening of a resonant mode can be reversed if the scattering of the radiating phonons becomes so strong that they are coherently trapped (localized). 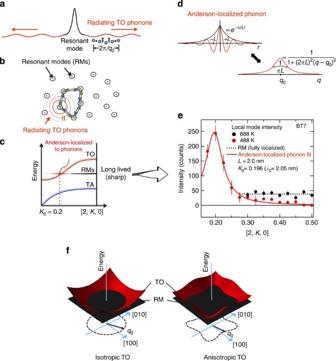Figure 4: Resonance modes coherently trapping ferroelectric modes. (a) Single resonance mode (RM) radiating energy through the TO phonon with which it is in resonance. (b) Anderson localization scheme for ferroelectric TO phonons eminating from and then scattered by resonance modes. Because they remain in phase, radiating ferroelectric phonons following two equal but opposite scattering paths (I, II) constructively interfere on returning to the source, which tends to coherently trap waves in disordered systems35. (c) Modification to the dispersion curves from an Anderson-localized standing TO phonon at the resonance wave vector. (d) Phonons trapped via Anderson localization at the resonance decay in real space exponentially with a localization lengthL, which transforms in reciprocal space to aq-space convolution of the phonon peak atq0with a Lorenztian width 1/πL(full-width at half-maximum). (e) Local mode intensities versusQ=[2,K, 0]. At 688 K the local mode intensity is flat, which is consistent with a fully localized resonance mode. At 488 K (red points), a Lorenztian function fit (red line) to the data results inL=2.0±0.2 nm andK0=0.196±0.005 (which is at the TO resonance crossing), a form consistent with Anderson-localized TO phonons. Local mode intensities (peak areas) were determined from peak fits to the data inFigs 1and2(seeSupplementary Fig. 6for details). (f) Effect of anisotropy in the TO phonon (red surfaces) on the trapping wave vectors,q0, determined by the intersection of the TO phonon surface with the resonance mode (black surface). Figure 4a shows a resonance mode radiating energy in the form of ferroelectric TO phonons at the resonance wave vector, q 0 . Arranging these randomly in 3D allows for the coherent trapping of phonons at the resonance via Anderson localization [32] , [33] , [34] , [35] , Fig. 4b . In the dispersion curves, such ferroelectric standing phonons, which are spatially localized standing TO modes at the resonance mode frequency, should result in a size broadening of the TO mode in q -space centred at the resonance wave vector, q 0 . Figure 4c illustrates how forming Anderson-localized ferroelectric phonons augments the spectrum. This explains the intensity shifting towards the resonance crossing in Figs 1c and 2a , as well as the absence of anticrossing effects, since a q -space broadening of the localized standing TO phonon is not a real crossing. The disappearance of the flat resonance mode intensity profile is also expected since the resonance modes become coherently bound to the Anderson-localized phonons, which causes them to lose their fully localized incoherent character. Figure 4: Resonance modes coherently trapping ferroelectric modes. ( a ) Single resonance mode (RM) radiating energy through the TO phonon with which it is in resonance. ( b ) Anderson localization scheme for ferroelectric TO phonons eminating from and then scattered by resonance modes. Because they remain in phase, radiating ferroelectric phonons following two equal but opposite scattering paths (I, II) constructively interfere on returning to the source, which tends to coherently trap waves in disordered systems [35] . ( c ) Modification to the dispersion curves from an Anderson-localized standing TO phonon at the resonance wave vector. ( d ) Phonons trapped via Anderson localization at the resonance decay in real space exponentially with a localization length L , which transforms in reciprocal space to a q -space convolution of the phonon peak at q 0 with a Lorenztian width 1/ πL (full-width at half-maximum). ( e ) Local mode intensities versus Q =[2, K , 0]. At 688 K the local mode intensity is flat, which is consistent with a fully localized resonance mode. At 488 K (red points), a Lorenztian function fit (red line) to the data results in L =2.0±0.2 nm and K 0 =0.196±0.005 (which is at the TO resonance crossing), a form consistent with Anderson-localized TO phonons. Local mode intensities (peak areas) were determined from peak fits to the data in Figs 1 and 2 (see Supplementary Fig. 6 for details). ( f ) Effect of anisotropy in the TO phonon (red surfaces) on the trapping wave vectors, q 0 , determined by the intersection of the TO phonon surface with the resonance mode (black surface). Full size image This interpretation is supported quantitatively by noting that Anderson localization is exponential [32] , [33] , [34] , [35] and, as illustrated in Fig. 4d , exponential localization of a phonon in real space transforms in reciprocal space to a q -space convolution of the phonon at the resonance wave vector, q 0 =(2 π / a ) K 0 , with a Lorentzian function ( a =lattice parameter). To separate the intensity of the localizing mode from the TO phonon, peak areas from fits to the data in Figs 1b,c and 2a,b are used (for fitting details see Supplementary Fig. 6 ). As shown in Fig. 4e , the Lorenztian function fits the q -dependence of the localizing mode intensity at 488 K with a least squares refinement giving a resonance wave vector K 0 =0.196±0.005, confirming a centre at the TO mode crossing, and a coherence length L =2.0±0.2 nm, which equals one resonance wavelength, λ 0 =2 π / q 0 = a / K 0 =2.05±0.05 nm. The match between the coherence length and the wavelength supports the notion of coherently trapped phonons. This profile is distinct from the flat profile at 688 K ( Fig. 4e ), where flat is consistent with fully localized resonance modes. Hence, on cooling to 488 K, fully localized resonance modes transform to long-lived (sharp in energy) standing (dispersionless) TO phonons (peak centre) that are limited to ~2 nm regions (profile in q ), occur at a frequency occupied by disordered resonant scatterers, and at a wavelength matching their size. These are hallmarks of Anderson-localized waves [32] , [33] , [34] , [35] . Given that the coherence length and wavelength of the Anderson-localized ferroelectric phonons match the known PNR coherence length [7] , that localization coincides with PNR formation and that such trapped ferroelectric modes induce electric polarization strongly suggests that these are the dynamical precursors to the PNRs. Further support for this connection can be found in the anistropy of the PNRs. To explain the correlation between anisotropy in the PNR diffuse scattering and the TO phonon in PMN- x PT (0< x <30%), Matsuura et al. [7] speculated that TO phonons might be trapped by PNRs, but did not explain how. Figure 4f illustrates how anisotropy in the TO phonon dispersion surface—as it intersects the resonance mode—projects anisotropy onto the resonance wave vector. For PMN-30%PT, the TO phonon is essentially isotropic [7] (as can be verified with our crystal, see Fig. 3a,c ), which produces isotropic ferroelectric mode trapping (left in Fig. 4f ), thus explaining isotropic PNRs [7] . For PMN, the TO phonon is ~20% softer along [110] than [100] [7] , which shifts the resonance wave vector to larger values along [110], resulting in an anisotropic butterfly shaped pattern (right in Fig. 4f ) that matches the anisotropic PNR diffuse scattering pattern in both size and shape [7] . The competing antiferroelectric distortions observed near the zone edges of PMN [17] might also be initiated by this mechanism. As shown in Fig. 3c , the only other place in the scattering plane where the TO mode crosses resonance mode frequency is at the M points on the zone edges, which could localize antiferroelectric TO modes at these points. Indeed, as shown in Figs 2c and 3f , a similar enhancment of the sharp localizing mode intensity occurs at the crossing near the M point on cooling from 688 to 488 K, consitent with the localization of a narrow band of antiferroelectric TO modes near these points. The fact that the localized mode intensity is less strongly peaked at the second crossing, compare Fig. 2a,c , is also consistent with antiferroelectric mode trapping since phonons near the zone edges have shorter wavelengths; singly trapped shorter wavelengths are smaller in real space and consequently broader in reciprocal space. For Anderson-localized ferroelectric phonons to explain the more intense diffuse scattering patterns and enhanced dielectric properties of relaxors, they must slow down. As the frequency of phonons decrease (slow), the mean square amplitudes (< u 2 >~ kT /(M ω 2 )) and scattering intensities grow as the inverse square of frequency, resulting in more intense scattering near the elastic line. Similarly, the Lyddane–Sachs–Teller relation indicates that the static dielectric contribution from the localized ferroelectric phonons will grow as the inverse square of its frequency. As mentioned above, such a slowing process has been explained in terms of the nonlinear dynamics of ILMs [25] , [26] , [27] . To explain the slowing of Anderson-localized phonons, we propose that on cooling, nonlinearity causes a growing subset of the Anderson-localized phonons to become ILM-like and slow down to form PNRs. Such a mechanism is supported by calculations showing that by varying the degrees of nonlinearity and disorder it is possible to change continuously between Anderson-localized modes (disorder localization) and ILMs (nonlinear localization), and these tend to localize at the same site [37] . This is in essence a competition between ILM and Anderson localization length scales [38] . In relaxors, inhomogeneous soft nonlinearity increases on cooling [25] , [26] , [27] , which can slow a subset of the Anderson-localized modes via ILM nonlinear slowing. The resulting distribution of slowing frequencies would map to the ILM models of relaxor ferroelectrics [25] , [26] , [27] , but the size, shape and distribution of the PNRs would be dictated by the resonance wave vector of the intiating Anderson-localized phonons. In this model, the vertical columns of diffuse inelastic intensity observed near the zone centre [14] and zone edges [17] are interpreted as the distribution of slowing local modes [25] , [26] , [27] . Additional neutron scattering measurements performed on (Pb(Zn 1/3 Nb 2/3 )O 3 ) 0.95 -(PbTiO 3 ) 0.05 (PZN-5%PT) using angular-range chopper spectrometer (ARCS) suggest that this phonon localization mechanism is not special to PMN-PT. As shown in Supplementary Fig. 7 , at 688 K a similar localized phonon feature appears between the TA and TO phonons in PZN-5%PT at about 10 meV, which is about 1.8 meV lower than that in PMN-30%PT at the same temperature. A lower energy local mode results in a crossing with the TO mode at a position closer to the zone centre. This is consistent with the PZN-PT system, which has a narrower region of PNR diffuse elastic scattering (larger PNRs) and a narrower phonon ‘waterfall’ [14] when compared with PMN-PT. Interestingly, independent concurrent studies to ours have been published very recently by Sherrington [20] , [39] in which Anderson localization as the origin of PNRs is derived theoretically, lending further independent support to the picture. To establish causality, it is worth considering the opposing argument that PNRs drive phonon localization rather than phonon localization drives PNRs. A simple counterargument to this idea is that phonon localization must lead because it develops 200 K above the stability limit of the PNRs ( Fig. 1 ). However, the complex pattern of localization provides for several additional counterarguments. To demonstrate this, let us assume hypothetically that PNR formation is driven by some other mechanism and that the TO phonons at wavelengths matching the size of the PNRs become trapped within the ‘structural’ PNRs, which would explain the observed PNR-sized localized ferroelectric mode feature at 488 K. Now consider what happens on heating from 488 to 688 K. From the structure factor of the localizing mode we see that the mode develops a flat intensity profile, which implies full localization. Hence, if the PNR size was dictating the local mode size, this would imply that the PNRs become much smaller with increasing temperature, but from diffuse scattering measurements we know that they do not, they stay about the same size [7] (which is expected for the Anderson localization picture since the trapping wave vector does not change much). Second, consider the relationship between the PNR diffuse scattering and TO phonon anisotropy. For this relationship to be maintained, the anisotropy of the PNRs would have to follow the anisotropy in the TO phonon dispersion in just such a way that the trapped wavelengths remain at a single frequency. If the anisotropy of the TO phonon increased but the PNRs did not change shape accordingly, then the trapped phonons would have to vary in frequency for the trapped wave vectors to match the same PNR size in different directions (see Fig. 4f ). Third, consider the corresponding antiferroelectric distortions. We see that these occur at the zone edges and that there is a local mode trapped at the same frequency ( Figs 3f and 2c ). If these phonon modes were also similarly trapped by antiferroelectric distortions, it is expected that their wave vectors would also match the size of the antiferroelectric distortions. For the frequencies to again match would require that the size of the antiferroelectric regions just happen to be such that they trap wave vectors at the zone edge that are at the same frequency as the phonons trapped at the zone centre and in multiple directions. This seems highly unlikely. Abandoning the notion that the frequency (dynamics) is the driver requires an implausible list of coincidences for the sizes/structure factors of the static features to be such that just a single frequency results. For all of these reasons we conclude that the phonon localization must drive the local structure, and not the other way around. In the picture that emerges from our measurements, T d is the temperature where localized resonance modes form on cooling towards the ferroelectric instability, most likely due to off-centring Pb atoms [31] . High-frequency PNRs are then generated by the trapping of single-wavelength ferroelectric phonons within the disordered resonance modes via Anderson localization [32] , [33] , [34] , [35] . The wave vector where the resonance mode crosses the ferroelectric phonon determines the size and shape of the PNRs, as well as competing antiferroelectric distortions at the zone edges [17] . The slowing of the PNRs is explained in terms of slowing Anderson-localized modes by the nonlinear ILM mechanism [25] , [26] , [27] . Without the formation of polar regions, relaxor ferroelectric behaviour would not occur. Hence, our results indicate that ferroelectric phonon localization plays a central role in relaxor ferroelectric behaviour. Triple-axis inelastic neutron scattering A 200-g plate-shaped (5 mm thick) single crystal of PMN-30%PT with the [100] crystallographic direction normal to the large face was measured using the bt7 triple-axis spectrometer at the NIST Center for Neutron Research [40] . At 5 mm thick, the crystal scatters ~20% of the neutrons at normal incidence. The spectrometer was operated with filtered fixed final neutron energy of 13.7 meV and the crystal was mounted in a furnace with the (hk0) reflections in the scattering plane using a vanadium holder. Measurements were made along [2, K , 0] at 21 equally spaced values of K between 0 and 0.5 for temperatures of 293, 488, 688 and 883 K. Additional temperatures were measured for K =0.15 and 0.2. To rule out spurious peaks as a source for the phonon localization feature, the spectral features were confirmed with measurements at equivalent points in reciprocal space. Spurious features, or spurions, may occur in triple-axis inelastic neutron scattering measurements due to higher order reflections from the monochromator or analyser, incoherent scattering from the monochromator or analyser and scattering from materials in the beam other than the crystal [41] . This type of scattering usually produces features in limited regions of reciprocal space, but in rare cases can produce streaks that mimic dispersion. Even in such cases, however, spurions are not expected to be temperature dependent and are also not expected to appear the same way in different equivalent parts of reciprocal space. Supplementary Fig. 2 shows constant Q scans taken at two equivalent Q points and at two different temperatures. The localizing mode around 12 meV appears similar in both cases and it has the same strong temperature dependence on heating from 688 K to around 900 K. This is inconsistent with spurious scattering. Furthermore, a calculation using Scan Mapper in the Data Analysis and Visualization Environment (DAVE) software [42] does not indicate any common spurious processes at this energy under these scattering conditions. In addition, the false-peak conditions for higher order harmonics for fixed E f =13.7 meV calculated up to fourth order produce no peak at +12 meV (also calculated in DAVE). Supplementary Table 1 lists these false-peak conditions. To further exclude the possibility that the localizing mode feature discussed in this manuscript is a technique-specific artefact, its existence was also confirmed using the ARCS TOF as discussed below. Supplementary Fig. 3 shows a comparison of results near the same Q point in reciprocal space. The features agree to within the error in the peak-fit positions. Multiphonon scattering also occurs but can be dismissed as an explanation for the sharp localizing mode for at least two reasons. First, multiphonon processes cannot produce peaks that are sharper than 1-phonon peaks. Even for sharp 1-phonon features, all the 2-phonon combinations with the other modes result in very broad 2-phonon scattering in both energy and momentum [43] . Second, multiphonon scattering should increase more rapidly with temperature than the 1-phonon scattering, yet in some locations the localizing mode actually decreases intensity with increasing temperature. While for the Q =(2, ±0.4, 0) data sets shown in Supplementary Fig. 2 the relative intensity of the localizing mode clearly increases with temperature, a decrease in relative intensity is observed nearby at Q =(2, 0.325, 0), as shown in Supplementary Fig. 4 . This is part of the more complex intensity behaviour described in the text, where intensity shifts from the zone boundary towards the zone centre, and is inconsistent with multiphonon scattering. TOF inelastic neutron scattering Additional measurements were performed on the same crystal using the ARCS at the Spallation Neutron Source of Oak Ridge National Laboratory [44] . Measurements were performed with the crystal oriented in the (hk0) plane and with an incident neutron energy of 25 meV. Comprehensive 4D Q -E volumes of data were obtained at 488 and 688 K, by rotating the angle between the [100] axis and the incident beam in 0.5° steps, collecting data at each angle from 0 to 60 °C and combining the data using MSlice in the Data Analysis and Visualization Environment (DAVE) software [42] . Additional measurements on a large (~100 g) single crystal of (Pb(Zn 1/3 Nb 2/3 )O 3 ) 0.95 -(PbTiO 3 ) 0.05 (PZN-5%PT) heated to 688 K were also performed on ARCS. The same crystal orientation and angle rotations were used for PZN-5%PT as described above for PMN-30%PT. X-ray characterization of the PMN-30%PT crystal Lattice thermal expansion was measured by X-ray diffraction. The sample was attached to a Mo thermal susceptor using Ag paint. A radiative electrical heater was used to heat this susceptor. Temperature was measured and controlled to within 0.1 K using a type K thermocouple attached to the sample using Ag paint. The sample was held in vacuum under a hemispherical Be X-ray window. Cu K X-rays generated by a Rigaku RU-300 rotating anode generator were monochromated by a sagittally bent graphite (0002) crystal, collimated by slits, scattered from the (100) face of the sample, collimated again by söller slits and counted by a NaI scintillation detector. Theta/2-theta scans were taken through the (200), (220) and (222) reflections as temperature was cycled between room temperature and 873 K. Lattice expansion was determined from Bragg’s law, with 2-theta found by fitting these scans to a Kα 1 / Kα 2 doublet of Gaussian peaks. Diffractometer angles were calibrated using the 0.5431, nm lattice parameter of a Si wafer. Crystals Large PMN-30%PT and PZN-5%PT crystals were grown by TRS technologies( http://www.trstechnologies.com/Materials/single_crystals.php ). How to cite this article: Manley, M. E. et al. Phonon localization drives polar nanoregions in a relaxor ferroelectric. Nat. Commun. 5:3683 doi: 10.1038/ncomms4683 (2014).